Genetics and the environment converge to dysregulateN-glycosylation in multiple sclerosis How environmental factors combine with genetic risk at the molecular level to promote complex trait diseases such as multiple sclerosis (MS) is largely unknown. In mice, N -glycan branching by the Golgi enzymes Mgat1 and/or Mgat5 prevents T cell hyperactivity, cytotoxic T-lymphocyte antigen 4 (CTLA-4) endocytosis, spontaneous inflammatory demyelination and neurodegeneration, the latter pathologies characteristic of MS. Here we show that MS risk modulators converge to alter N -glycosylation and/or CTLA-4 surface retention conditional on metabolism and vitamin D 3 , including genetic variants in interleukin-7 receptor-α ( IL7RA *C), interleukin-2 receptor-α ( IL2RA *T), MGAT1 (IV A V T−T ) and CTLA-4 (Thr17Ala). Downregulation of Mgat1 by IL7RA *C and IL2RA *T is opposed by MGAT1 (IV A V T−T ) and vitamin D 3 , optimizing branching and mitigating MS risk when combined with enhanced CTLA-4 N -glycosylation by CTLA-4 Thr17. Our data suggest a molecular mechanism in MS whereby multiple environmental and genetic inputs lead to dysregulation of a final common pathway, namely N -glycosylation. Multiple sclerosis (MS) is an autoimmune and neurodegenerative disorder influenced by genetics, female gender and vitamin D 3 (refs 1 , 2 , 3 ). Molecular mechanisms demonstrating how gene–gene and gene–environmental interactions combine to regulate disease risk remain largely unknown. Genome-wide association studies (GWAS) of common polymorphisms have identified only a proportion of the genetic variation responsible for familial disease clustering in complex trait diseases such as MS [4] , leading some to suggest that rare and highly penetrant variants account for the missing heritability [5] , [6] , [7] , [8] . However, rare and highly penetrant variants often display Mendelian type inheritance and are relatively insensitive to environmental influences (for example, cystic fibrosis). An alternative is epistatic interactions [9] between multiple independent alleles and the environment that affect a common biochemical pathway, whereby each factor has only a minor genetic and/or biological effect, but when combined results in severe deficiencies. Consistent with this, MS concordance rates in monozygotic twins are only ∼ 30% (ref. 10 ), despite recent evidence that discordant twins do not harbour significant sequence differences in their genome, epigenome and transcriptome [11] . This implies direct environmental impact on genetic risk. Virtually all cell surface and secreted proteins in metazoans are modified by co- and/or post-translational addition of complex carbohydrates in the endoplasmic reticulum/Golgi secretory pathway [12] , [13] , providing information encoding distinct from the genome [14] . Unlike DNA/RNA/protein, production of complex carbohydrates is not template driven, but rather is controlled by the activity of endoplasmic reticulum/Golgi enzymes and metabolic supply of their substrates. The branching and number of N- glycans per protein molecule cooperate to regulate binding to galectins, forming a molecular lattice at the cell surface that controls the concentration and endocytosis of surface glycoproteins [14] . N -Glycan number is gene-encoded while branching is conditional to activity of the Golgi α-mannosidases, N -acetylglucosaminyltransferases I, II, IV and V (Mgat1, 2, 4 and 5) and hexosamine pathway production of the substrate uridine diphosphate N -acetylglucosamine (UDP-GlcNAc) [15] , [16] ( Fig. 1a ). In mice, genetic deficiencies in N -glycan branching promote neurodegeneration, spontaneous inflammatory demyelination, T cell receptor (TCR) clustering/signalling, T helper 1 (T H 1) differentiation and endocytic loss of the growth and autoimmune inhibitor cytotoxic T-lymphocyte antigen 4 (CTLA-4), phenotypes that can be reversed by metabolic supplementation to UDP-GlcNAc biosynthesis [15] , [16] , [17] , [18] , [19] , [20] , [21] . 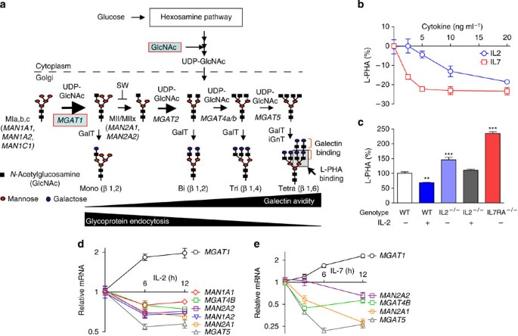Figure 1: IL-2 and IL-7 signalling regulateN-glycan branching in T cells. (a) Hexosamine andN-glycan branching pathway in mammals. Medial Golgi enzymes Mgat1, 2, 4a/b, and 5 generate mono-, bi-, tri- and tetra-antennary branchedN-glycans, respectively, in a sequential manner that is dependent on the supply of a common substrate, UDP-GlcNAc. GlcNAc branches are further modified to createN-acetyllactosamine units, which serve as binding sites for galectins andL-PHA. Mgat1, 2, 4 and 5,N-acetylglucosaminyltransferases I, II IV and V; MII/MIIx, mannosidase II/IIx, MIa,b,c, mannosidase I,a,b,c; SW, swainsonine. Additional structural diversity by addition of sialic acid, fucose,N-acetylgalactosamine and/or sulphate is not shown12. (b) Resting human PBMCs were treated for 3 days as indicated and analysed forL-PHA binding by fluorescence-activated cell sorting, gating on CD4+CD25−resting populations based on forward versus side scatter. MFI for control cells was used to normalize data. (c) Resting mouse splenocytes with the indicated genotypes were treated with IL-2 (20 ng ml−1) and analysed as inb. (d) Quantitative reverse transcription PCR on cDNA derived from resting human CD3+T cells treated with IL-2 (20 ng ml−1) in triplicate. (e) Resting Human PBMCs were treated with IL-7 (20 ng ml−1) and analysed as ind. Genotypes for human cells wereIL2RA*TC andIL7RA*CC except ford, which wasIL2RA*TT.Pvalues by analysis of variance and the Newman–Keuls Multiple Comparison Test. ***P<0.001, **P<0.01 in all panels. Error bars are standard error of triplicate or greater values in all panels. Figure 1: IL-2 and IL-7 signalling regulate N -glycan branching in T cells. ( a ) Hexosamine and N -glycan branching pathway in mammals. Medial Golgi enzymes Mgat1, 2, 4a/b, and 5 generate mono-, bi-, tri- and tetra-antennary branched N -glycans, respectively, in a sequential manner that is dependent on the supply of a common substrate, UDP-GlcNAc. GlcNAc branches are further modified to create N -acetyllactosamine units, which serve as binding sites for galectins and L -PHA. Mgat1, 2, 4 and 5, N -acetylglucosaminyltransferases I, II IV and V; MII/MIIx, mannosidase II/IIx, MIa,b,c, mannosidase I,a,b,c; SW, swainsonine. Additional structural diversity by addition of sialic acid, fucose, N -acetylgalactosamine and/or sulphate is not shown [12] . ( b ) Resting human PBMCs were treated for 3 days as indicated and analysed for L -PHA binding by fluorescence-activated cell sorting, gating on CD4 + CD25 − resting populations based on forward versus side scatter. MFI for control cells was used to normalize data. ( c ) Resting mouse splenocytes with the indicated genotypes were treated with IL-2 (20 ng ml −1 ) and analysed as in b . ( d ) Quantitative reverse transcription PCR on cDNA derived from resting human CD3 + T cells treated with IL-2 (20 ng ml −1 ) in triplicate. ( e ) Resting Human PBMCs were treated with IL-7 (20 ng ml −1 ) and analysed as in d . Genotypes for human cells were IL2RA *TC and IL7RA* CC except for d , which was IL2RA *TT. P values by analysis of variance and the Newman–Keuls Multiple Comparison Test. *** P <0.001, ** P <0.01 in all panels. Error bars are standard error of triplicate or greater values in all panels. Full size image In this study, we investigate whether similar mechanisms are active in MS through detailed biological characterization of known polymorphisms and a unique candidate gene approach. Our data suggests that N -glycosylation provides the first unifying molecular mechanism in MS, whereby convergent genetic dysregulation is modulated by multiple environmental inputs such as metabolism and sunlight/vitamin D 3 . IL-2 and IL-7 regulate T cell growth via N -glycan branching Interleukin-2 receptor ( IL-2R ) and interleukin-7 receptor (IL-7R) are members of the common γ chain cytokine receptor family and use signal transduction through Stat5. Recently, genetic alterations in the IL-2 and IL-7 signalling pathways have been implicated in MS [3] , [22] , [23] . To examine whether these pathways alter N -glycan branching, we used flow cytometry with L -PHA ( Phaseolus vulgaris , leukoagglutinin), a plant lectin that binds specifically to β1,6GlcNAc-branched N -glycans, the product of Mgat5 ( Fig. 1a ) [18] , [24] . Addition of exogenous IL-2 or IL-7 to resting human T cells reduced L -PHA-binding structures (hereafter termed as branching) in CD25 − CD4 + T cells by ∼ 20–30% ( Fig. 1b and Supplementary Fig. S1a ). Analysis of IL-2 and IL-7RA deficient ex vivo CD25 − CD4 + mouse T cells revealed ∼ 50% and >2-fold increases in branching, respectively, confirming that autocrine IL-2 and IL-7 signalling regulates branching in vivo ( Fig. 1c ). As ∼ 15–20% change in L -PHA binding is sufficient to alter T cell function, growth and autoimmune risk [16] , [20] , these alterations are highly significant and in the case of IL-7RA deficiency, represents the largest change observed outside of direct manipulation of the Golgi branching pathway. Indeed, addition of exogenous IL-2 or IL-7 both induce ∼ 2-fold increase in the Golgi MGAT1 mRNA as well as ∼ 1.5–3-fold decreases in Golgi MGAT5 , MGAT4B , mannosidase II and IIx ( MAN2A1 , MAN2A2 ) and mannosidase Ia and b ( MAN1A1 , MAN1A2 ; Fig. 1d,e ). These mRNA changes are opposite of that induced by TCR signalling, which enhances branching [25] . Mgat1 has a ∼ 250-fold higher affinity for UDP-GlcNAc than Mgat5 and over expression of Mgat1, particularly in the presence of reduced Mgat4 and Mgat5, decreases branching by limiting UDP-GlcNAc supply to Mgat4 and Mgat5 (refs 15 , 25 ). T cell activation enhances branching as well as IL-2 and IL-2RA expression; therefore, we next examined the effects of IL-2 and IL-7 signalling in T cell blasts. Exogenous IL-2 enhanced TCR signalling-induced increases in branching in CD25 + CD4 + mouse and human T cell blasts, whereas anti-IL-2 neutralizing antibody, the IL-2RA antagonist Ro26-4550 and/or IL-2 deficiency had the opposite effect ( Fig. 2a and Supplementary Fig. S1b ). Similarly, addition of exogenous IL-7 increased branching in human CD25 + CD4 + T cell blasts, whereas deficiency of IL-7RA limited upregulation of branching in mouse CD25 + CD4 + T cell blasts ( Fig. 2b and Supplementary Fig. S1b ). IL-2 treatment significantly enhanced transcripts of MGAT1 > MAN2A2 > MGAT5 in TCR-activated CD25 + CD3 + T cells ( Supplementary Fig. S1c ). These data are consistent with the ultra-sensitive kinetics of the Golgi branching pathway [15] , in which MGAT1 hyperactivity limits branching in resting T cells with low UDP-GlcNAc and Mgat5 activity, but enhances branching in T cell blasts where UDP-GlcNAc, Mgat5 and mannosidase IIx are enhanced. CD25 is also constitutively expressed by FoxP3 + T regulatory cells; however, IL-2 enhanced branching to a much greater extent in CD25 + FoxP3 − T cell blasts ( Supplementary Fig. S1d ). Thus, IL-2 and IL-7 co-regulate multiple Golgi genes to reduce branching in resting T cells; but promote branching in T cell blasts. 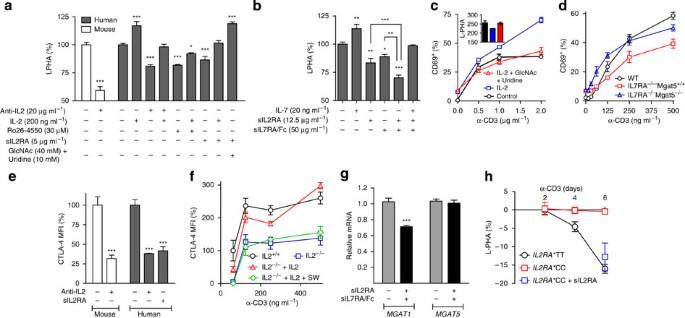Figure 2:IL2RA*T andIL7RA*C MS risk alleles limitN-glycan branching in T cell blasts. (a) Human CD3+T cells or mouse splenocytes were stimulated with anti-CD3 (200 ng ml−1) and treated as indicated for 5 days. CD25+CD4+T cell blasts were analysed forL-PHA binding by fluorescence-activated cell sorting (FACS). Ro26-4550 is an IL-2RA antagonist. (b) Human T cells were stimulated with anti-CD3 (200 ng ml−1) and treated as indicated for 5 days. CD25+CD4+T cell blasts were analysed as ina. (c) Purified human T cells were pre-treated for 3 days with IL-2 (20 ng ml−1) and/or GlcNAc (40 mM)+uridine (10 mM), and then stimulated with anti-CD3 for 24 h. CD4+T cells were analysed for CD69 expression andL-PHA binding by FACS. (d) Mouse splenocytes with the indicated genotypes were stimulated with anti-CD3 for 24 h. CD4+ T cells were analysed as inc. (e) Human T cells or mouse splenocytes were stimulated with anti-CD3 (200 ng ml−1) and treated with anti-IL2 (20 μg ml−1) or sIL2RA (5 μg ml−1) for 5 days. CD25+CD4+T cell blasts were analysed for CTLA-4 surface expression. Data are normalized to control and by subtracting background from unstimulated CD4+T cells. (f) Mouse splenocytes with the indicated genotypes were stimulated with anti-CD3 for 5 days, with or without IL-2 (20 ng ml−1) and/or SW (150 nM) addition at day 3. CD25+CD4+T cell blasts were analysed for CTLA-4 surface expression as ine. (g) Human CD25+CD4+T cells were stimulated with anti-CD3 (200 ng ml−1) and treated with sIL2RA (12.5 μg ml−1) and/or sIL7RA/Fc (50 μg ml−1) for 3 days. Relative mRNA levels were measured by quantitative reverse transcription PCR (normalized to actin). (h) Human T cells (IL7RA*CC) with the indicated genotypes were stimulated with anti-CD3 (200 ng ml−1) for 2–6 days, with or without sIL2RA (12.5 μg ml−1). CD25+CD4+T cell blasts were analysed forL-PHA binding by FACS as ina. Genotypes wereIL2RA*CC andIL7RA*CC ina;IL2RA*CT andIL7RA*CT inb,eandg;IL2RA*CT andIL7RA*CT incandd; all lacked theMGAT1IVAVT−Thaplotype.Pvalues by analysis of variance and the Newman–Keuls Multiple Comparison Test. ***P<0.001, **P<0.01, *P<0.05 in all panels. Error bars are standard error of triplicate or greater values in all panels. Figure 2: IL2RA* T and IL7RA* C MS risk alleles limit N -glycan branching in T cell blasts. ( a ) Human CD3 + T cells or mouse splenocytes were stimulated with anti-CD3 (200 ng ml −1 ) and treated as indicated for 5 days. CD25 + CD4 + T cell blasts were analysed for L -PHA binding by fluorescence-activated cell sorting (FACS). Ro26-4550 is an IL-2RA antagonist. ( b ) Human T cells were stimulated with anti-CD3 (200 ng ml −1 ) and treated as indicated for 5 days. CD25 + CD4 + T cell blasts were analysed as in a . ( c ) Purified human T cells were pre-treated for 3 days with IL-2 (20 ng ml −1 ) and/or GlcNAc (40 mM)+uridine (10 mM), and then stimulated with anti-CD3 for 24 h. CD4 + T cells were analysed for CD69 expression and L -PHA binding by FACS. ( d ) Mouse splenocytes with the indicated genotypes were stimulated with anti-CD3 for 24 h. CD4+ T cells were analysed as in c . ( e ) Human T cells or mouse splenocytes were stimulated with anti-CD3 (200 ng ml −1 ) and treated with anti-IL2 (20 μg ml −1 ) or sIL2RA (5 μg ml −1 ) for 5 days. CD25 + CD4 + T cell blasts were analysed for CTLA-4 surface expression. Data are normalized to control and by subtracting background from unstimulated CD4 + T cells. ( f ) Mouse splenocytes with the indicated genotypes were stimulated with anti-CD3 for 5 days, with or without IL-2 (20 ng ml −1 ) and/or SW (150 nM) addition at day 3. CD25 + CD4 + T cell blasts were analysed for CTLA-4 surface expression as in e . ( g ) Human CD25 + CD4 + T cells were stimulated with anti-CD3 (200 ng ml −1 ) and treated with sIL2RA (12.5 μg ml −1 ) and/or sIL7RA/Fc (50 μg ml −1 ) for 3 days. Relative mRNA levels were measured by quantitative reverse transcription PCR (normalized to actin). ( h ) Human T cells ( IL7RA *CC) with the indicated genotypes were stimulated with anti-CD3 (200 ng ml −1 ) for 2–6 days, with or without sIL2RA (12.5 μg ml −1 ). CD25 + CD4 + T cell blasts were analysed for L -PHA binding by FACS as in a . Genotypes were IL2RA *CC and IL7RA* CC in a ; IL2RA *CT and IL7RA* CT in b , e and g ; IL2RA *CT and IL7RA* CT in c and d ; all lacked the MGAT1 IV A V T−T haplotype. P values by analysis of variance and the Newman–Keuls Multiple Comparison Test. *** P <0.001, ** P <0.01, * P <0.05 in all panels. Error bars are standard error of triplicate or greater values in all panels. Full size image Cytokine-induced alterations in branching are expected to initially promote TCR-mediated growth [18] , followed by enhanced growth arrest of T cell blasts by increased CTLA-4 surface expression [15] . Indeed, pretreatment of resting human T cells with IL-2 significantly enhanced TCR signalling-mediated upregulation of CD69 in the absence but not presence of N -acetylglucosamine (GlcNAc) and uridine ( Fig. 2c ). GlcNAc and uridine enhance branching by increasing UDP-GlcNAc supply to the Golgi [15] , [16] , and rescued reductions induced by IL-2 ( Fig. 2c inset). Similarly, analysis of IL7RA −/− Mgat5 −/− double knockout mice revealed that suppression of TCR activation by IL7RA deficiency requires Mgat5 ( Fig. 2d ). In CD25 + CD4 + T cell blasts, anti-IL-2 neutralizing antibody and IL-2 deficiency reduced CTLA-4 surface expression ( Fig. 2e,f ), the latter reversed by the addition of exogenous IL-2 in the absence but not presence of swainsonine (SW; Fig. 2f ). SW is an inhibitor of Golgi α-mannosidase II/IIx that reduces branching downstream of Mgat1 ( Fig. 1a ) [26] , confirming that IL-2 promotes CTLA-4 surface retention by increasing branching. IL2RA and IL7RA MS risk alleles reduce MGAT1 and branching The IL2RA *T (rs2104286) and IL7RA *C (rs6897932) MS risk alleles are the common alleles in Caucasian populations (frequency ∼ 75%) and are associated with enhanced secretion of soluble receptors (that is, sIL2RA and sIL7RA) that bind cognate cytokines and antagonize signalling ( Supplementary Fig. S2a–c ) [22] , [27] , [28] , [29] . Exogenous sIL2RA and sIL7RA/Fc chimera both reduced branching in CD25 + CD4 + T cell blasts, an effect that was additive when combined and rescued by exogenous IL-7 or GlcNAc ( Fig. 2a,b ). Blocking IL-2 and IL-7 signalling with sIL2RA and sIL7RA or anti-IL-2 and anti-IL-7 neutralizing antibodies both reduced MGAT1 mRNA in CD25 + CD4 + T cell blasts, yet had little effect on MGAT5 expression ( Fig. 2g and Supplementary Fig. S2d ). sIL2RA reduced CTLA-4 surface levels in T cell blasts to a similar degree as anti-IL-2 neutralizing antibody ( Fig. 2e ). Directly comparing T cell blasts with or without the IL2RA *T risk allele revealed minimal differences in branching during early stages of activation; however by day 6, branching in IL2RA* TT and IL2RA* TC blasts was significantly reduced relative to IL2RA* CC blasts ( Fig. 2h , Supplementary Fig. S2e ), consistent with enhanced endogenous sIL2RA production by the T allele. Addition of exogenous sIL2RA to IL2RA* CC T cell cultures lowered branching at day 6 to that observed in IL2RA* TT blasts ( Fig. 2h ), confirming differences in branching arose from reduced endogenous sIL2RA in IL2RA* CC T cell cultures. Thus, soluble receptors associated with the IL2RA *T and IL7RA *C risk alleles combine to downregulate MGAT1 and branching in T cell blasts. MGAT1 variants alter branching conditional on metabolism Next, we directly screened the MGAT1 gene for functional variants. Sequencing the MGAT1 coding region (exon 2) in 42 MS patients identified a high frequency of variants suitable for functional testing ( Supplementary Fig. S3a ). The direct cloning of PCR-amplified genomic DNA revealed multiple haplotypes that rescued cell surface binding to L -PHA when transiently transfected into Lec1 cells [30] , an Mgat1-deficient Chinese Hamster Ovary cell line ( Fig. 3a and Supplementary Fig. S3b,c ). All variant haplotypes were less effective than the common haplotype, with those harbouring both the IV A (rs7726005) and V T−T (rs2070924 and rs2070925) polymorphisms reducing branching ∼ 20%. The IV A and V T−T polymorphisms seem to exert additive effects, as separately each displayed a ∼ 10% reduction in branching. Consistent with this, anti-CD3 and myelin-activated T cells heterozygous for the IV A and V T−T polymorphisms (hereafter referred as the MGAT1 IV A V T−T haplotype) displayed reduced upregulation of branching ( Fig. 3b,c ). Transient transfection into Lec1 cells demonstrated that the IV A , V T−T and IV A V T−T haplotypes increased Mgat1 activity ∼ 2-, 2- and 3-fold, respectively, a phenotype also associated with peripheral blood mononuclear cells (PBMCs) harbouring the MGAT1 IV A V T−T haplotype ( Fig. 3d,e ). Matrix-assisted laser desorption/ionization–time of flight mass spectroscopy confirmed the N -glycan product of Mgat1 (mono-antennary) was increased relative to its N -glycan acceptor (Man 5 GlcNAc 2 ) in PBMCs with the MGAT1 IV A V T−T haplotype ( Fig. 3f and Supplementary Fig. S3d ). 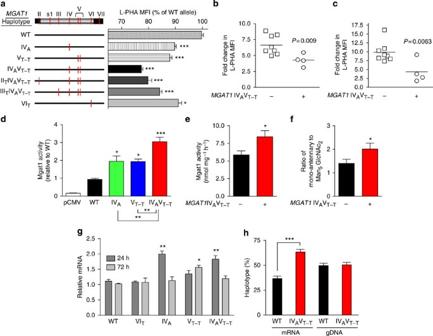Figure 3:MGAT1haplotypes reduceN-glycan branching. (a)MGAT1exon 2 was amplified by PCR from genomic DNA, cloned into the pCMV vector, sequenced to identify haplotypes, transiently transfected into Mgat1-deficient CHO cells (Lec1) in triplicate and analysed 3 days later byL-PHA fluorescence-activated cell sorting. MFI was determined on theL-PHA+population and normalized to the common haplotype (WT). (b) Anti-CD3 or (c) myelin peptide was used to stimulate PBMCs from healthy human controls for 48 h. Fold increase inL-PHA MFI in CD4+T cells following stimulation was determined by comparing unstimulated resting cells with blasting cells in each subject. All subjects had ≥3IL2RA*T+IL7RA*C risk alleles, except one subject in each group heterozygous for both. (d) Mgat1-deficient Lec1 cells were transiently transfected with the indicatedMGAT1haplotypes and lysed to assess Mgat1 enzyme activity. Average Mgat1 activity for WT (common haplotype) was 6.45 nmol mg−1h−1. Activities were normalized for transfection efficiency. (e) Human PBMCs with the indicated genotypes (n=4 per genotype) were lysed to assess Mgat1 enzyme activity as ind. Subjects had ≥3IL2RA*T+IL7RA*C risk alleles. (f)N-Glycans in human PBMCs with the indicated genotypes (n=6 per genotype) were analysed by matrix-assisted laser desorption/ionization–time of flight mass spectroscopy and normalized by taking the ratio of the intensity of mono-antennary ((Gal)GlcNAc1Man5GlcNAc2) to Man5GlcNAc2, the product and acceptor of Mgat1, respectively. Subjects had ≥3IL2RA*T+IL7RA*C risk alleles except for twoMGAT1IVAVT−Tsubjects that were double heterozygotes; removal of which does not alter the result (that is, 2.01 versus 1.97). (g) Lec1 cells transfected with the indicatedMGAT1haplotypes were analysed for relative mRNA levels by quantitative reverse transcription PCR. Expression was normalized for transfection efficiency. (h) Human PBMCs from two heterozygousMGAT1IVAVT−Tsubjects were examined for differential allelic expression by comparing the relative abundance of mRNA and genomic DNA (gDNA) for each haplotypein vivo.Pvalues inb,c,e,fandhbyt-test and panelsa,dandgby analysis of variance and the Newman–Keuls Multiple Comparison Test. *P<0.05, **P<0.01, ***P<0.001 in all panels. Error bars are standard error of triplicate or greater values in all panels. Figure 3: MGAT1 haplotypes reduce N -glycan branching. ( a ) MGAT1 exon 2 was amplified by PCR from genomic DNA, cloned into the pCMV vector, sequenced to identify haplotypes, transiently transfected into Mgat1-deficient CHO cells (Lec1) in triplicate and analysed 3 days later by L -PHA fluorescence-activated cell sorting. MFI was determined on the L -PHA + population and normalized to the common haplotype (WT). ( b ) Anti-CD3 or ( c ) myelin peptide was used to stimulate PBMCs from healthy human controls for 48 h. Fold increase in L -PHA MFI in CD4 + T cells following stimulation was determined by comparing unstimulated resting cells with blasting cells in each subject. All subjects had ≥3 IL2RA* T+ IL7RA* C risk alleles, except one subject in each group heterozygous for both. ( d ) Mgat1-deficient Lec1 cells were transiently transfected with the indicated MGAT1 haplotypes and lysed to assess Mgat1 enzyme activity. Average Mgat1 activity for WT (common haplotype) was 6.45 nmol mg −1 h −1 . Activities were normalized for transfection efficiency. ( e ) Human PBMCs with the indicated genotypes ( n =4 per genotype) were lysed to assess Mgat1 enzyme activity as in d . Subjects had ≥3 IL2RA* T+ IL7RA* C risk alleles. ( f ) N -Glycans in human PBMCs with the indicated genotypes ( n =6 per genotype) were analysed by matrix-assisted laser desorption/ionization–time of flight mass spectroscopy and normalized by taking the ratio of the intensity of mono-antennary ((Gal)GlcNAc 1 Man 5 GlcNAc 2 ) to Man 5 GlcNAc 2 , the product and acceptor of Mgat1, respectively. Subjects had ≥3 IL2RA* T+ IL7RA* C risk alleles except for two MGAT1 IV A V T−T subjects that were double heterozygotes; removal of which does not alter the result (that is, 2.01 versus 1.97). ( g ) Lec1 cells transfected with the indicated MGAT1 haplotypes were analysed for relative mRNA levels by quantitative reverse transcription PCR. Expression was normalized for transfection efficiency. ( h ) Human PBMCs from two heterozygous MGAT1 IV A V T−T subjects were examined for differential allelic expression by comparing the relative abundance of mRNA and genomic DNA (gDNA) for each haplotype in vivo . P values in b , c , e , f and h by t -test and panels a , d and g by analysis of variance and the Newman–Keuls Multiple Comparison Test. * P <0.05, ** P <0.01, *** P <0.001 in all panels. Error bars are standard error of triplicate or greater values in all panels. Full size image The MGAT1 IV A V T−T haplotype harbours three polymorphisms in exon 2: an upstream non-synonymous coding single-nucleotide polymorphism (SNP; IV A : G1164A encoding Arg223Gln) and two synonymous coding SNPs that are ten nucleotides apart (V T−T : C1637T and G1648T). On the basis of the Mgat1 enzyme crystal structure, Arg223Gln is a surface-exposed residue far from the active site and therefore unlikely to effect enzyme activity [31] . However, IV A increased MGAT1 mRNA levels relative to the common haplotype in Lec1-transfected cells ( Fig. 3g ). The two synonymous SNPs in V T−T , with or without IV A , also increased mRNA expression following transfection, although with differing kinetics. Analysis of heterozygous PBMCs confirmed mRNA levels of the MGAT1 IV A V T−T haplotype were ∼ 2-fold higher than the common haplotype in vivo ( Fig. 3h ). The Km of Mgat5 for UDP-GlcNAc is significantly higher than Mgat1 ( ∼ 11 versus ∼ 0.04 mM), whereas this difference is reversed for their respective N -glycan acceptors ( ∼ 0.087 versus ∼ 2 mM) [15] . The ∼ 2- to 3-fold increase in Mgat1 expression induced by the MGAT1 IV A V T−T haplotype increased Mgat1 product ( Fig. 3f ) while also reducing UDP-GlcNAc supply to downstream Mgat5. The latter is predicted to reduce β1,6GlcNAc branching by Mgat5, and indeed, this was observed both experimentally ( Fig. 3a,b ) and with computational modelling ( Fig. 4a ) [15] . Thus, MGAT1 IV A V T−T functions dominantly to reduce branching under basal UDP-GlcNAc levels, but with increasing UDP-GlcNAc and/or Mgat5 levels, enhanced Mgat1 expression is expected to become less effective in limiting supply of UDP-GlcNAc to Mgat5, thereby allowing Mgat5 to act on the increased supply of N -glycan acceptors from Mgat1 to first equalize and then super-rescue β1,6GlcNAc branching. Indeed, these pathway dynamics were revealed by computational modelling ( Supplementary Fig. S4a ) and confirmed experimentally by increasing UDP-GlcNAc levels in transiently transfected Lec1 cells and CD4 + T cells by GlcNAc supplementation ( Fig. 4b and Supplementary Fig. S4b ). Consistent with this model, the magnitude of super-rescue by GlcNAc for the IV A , V T−T and IV A V T−T haplotypes was proportional to baseline enzyme activities. Thus, the gain-of-function haplotypes of MGAT1 -reduce branching under basal conditions, but enhance levels when UDP-GlcNAc and/or Mgat5 are increased above a threshold. 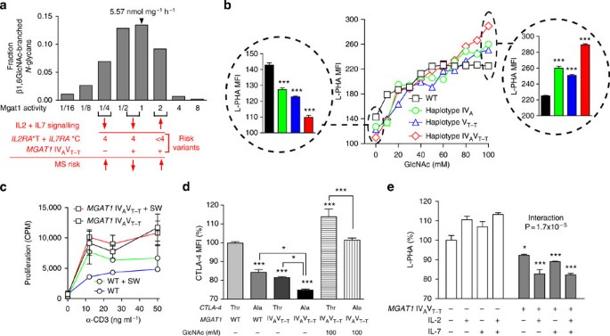Figure 4: Conditional regulation ofN-glycan branching and T cell growth byMGAT1IVAVT−T. (a) Ordinary differential equation model of medial Golgi enzyme reactions showing predicted alterations in β1,6GlcNAc branching when varying Mgat1 activity in the presence of fixed activities in Mgat2, 4 and 5. Activities in resting mouse 129/Sv T cells were used for Mgat1, Mgat2, Mgat5 (ref.20), whereas Mgat4 was estimated. In red, predicted effects of IL2/IL7 signalling and various genetic combinations ofIL2RA*T+IL7RA*Crisk alleles (four alleles or less than four) on Mgat1 activity, β1,6GlcNAc branching and MS risk in the absence or presence of theMGAT1IVAVT−Thaplotype. (b) Mgat1-deficient Lec1 cells transiently transfected as indicated were co-incubated with or without GlcNAc for 3 days and then analysed by fluorescence-activated cell sorting (FACS) forL-PHA binding.Pvalues by analysis of variance (ANOVA) and Newman–Keuls Multiple Comparison Test. (c) PBMCs heterozygous for theMGAT1IVAVT−Thaplotype (n=2 subjects assayed in triplicate) or homozygous for the common haplotype (WT;n=1 subject assayed in triplicate) were stimulated with anti-CD3 and analysed for proliferation as indicated for 2 days. Subjects used wereIL2RA*T/C,IL7RA*CC and CTLA-4 Thr/Ala. Error bars represent range of all values. (d) Transiently transfected Lec1 cells with or without GlcNAc treatment (3 days) were analysed for CTLA-4 expression by fluorescence-activated cell sorting.Pvalues by ANOVA and Newman–Keuls Multiple Comparison Test. (e) PBMCs with the indicated genotype (n=2) were stimulated with anti-CD3 (200 ng ml−1) and treated with IL-2 (20 ng ml−1) and IL-7 (20 ng ml−1) for 5 days. Subjects used wereIL2RA*T/C,IL7RA*CC and CTLA-4 Thr/Thr. Data is the average of triplicate values for each subject.Pvalues by 2-way ANOVA and Bonferoni's multiple comparison test. *P<0.05, **P<0.01, ***P<0.001 in all panels. Error bars are standard error of triplicate or greater values in all panels unless otherwise stated. Figure 4: Conditional regulation of N -glycan branching and T cell growth by MGAT1 IV A V T−T . ( a ) Ordinary differential equation model of medial Golgi enzyme reactions showing predicted alterations in β1,6GlcNAc branching when varying Mgat1 activity in the presence of fixed activities in Mgat2, 4 and 5. Activities in resting mouse 129/Sv T cells were used for Mgat1, Mgat2, Mgat5 (ref. 20 ), whereas Mgat4 was estimated. In red, predicted effects of IL2/IL7 signalling and various genetic combinations of IL2RA*T + IL7RA*C risk alleles (four alleles or less than four) on Mgat1 activity, β1,6GlcNAc branching and MS risk in the absence or presence of the MGAT1 IV A V T−T haplotype. ( b ) Mgat1-deficient Lec1 cells transiently transfected as indicated were co-incubated with or without GlcNAc for 3 days and then analysed by fluorescence-activated cell sorting (FACS) for L -PHA binding. P values by analysis of variance (ANOVA) and Newman–Keuls Multiple Comparison Test. ( c ) PBMCs heterozygous for the MGAT1 IV A V T−T haplotype ( n =2 subjects assayed in triplicate) or homozygous for the common haplotype (WT; n =1 subject assayed in triplicate) were stimulated with anti-CD3 and analysed for proliferation as indicated for 2 days. Subjects used were IL2RA* T/C, IL7RA* CC and CTLA-4 Thr/Ala. Error bars represent range of all values. ( d ) Transiently transfected Lec1 cells with or without GlcNAc treatment (3 days) were analysed for CTLA-4 expression by fluorescence-activated cell sorting. P values by ANOVA and Newman–Keuls Multiple Comparison Test. ( e ) PBMCs with the indicated genotype ( n =2) were stimulated with anti-CD3 (200 ng ml −1 ) and treated with IL-2 (20 ng ml −1 ) and IL-7 (20 ng ml −1 ) for 5 days. Subjects used were IL2RA* T/C, IL7RA* CC and CTLA-4 Thr/Thr. Data is the average of triplicate values for each subject. P values by 2-way ANOVA and Bonferoni's multiple comparison test. * P <0.05, ** P <0.01, *** P <0.001 in all panels. Error bars are standard error of triplicate or greater values in all panels unless otherwise stated. Full size image Consistent with reduced branching, resting PBMCs heterozygous for the MGAT1 IV A V T−T haplotype were more sensitive to TCR agonist than cells homozygous for the common MGAT1 haplotype ( Fig. 4c ). Blocking the branching with SW enhanced proliferation of cells with the common MGAT1 haplotype, but had little effect on cells heterozygous for the MGAT1 IV A V T−T haplotype, the latter consistent with the pre-existing deficiency in branching ( Fig. 4c ). The Thr17Ala polymorphism in human CTLA-4 encodes a non-synonymous SNP (49A/G, rs231775) in the signal peptide that reduces average N -glycan occupancy at the two N-X-S/T sites from two to one, limiting CTLA-4 surface levels and promoting T cell proliferation [32] , [33] . Such alterations in N -glycan number are expected to interact with the MGAT1 IV A V T−T haplotype to control CTLA-4 surface expression [15] . Indeed, computational modelling, co-transfection of Lec1 cells and analysis of T cell blasts confirmed previous observations [32] , [33] of significantly lower surface CTLA-4 Ala17 (that is, one N -glycan) compared with CTLA-4 Thr17 (that is, two N -glycans) when co-expressed with the common MGAT1 haplotype ( Fig. 4d and Supplementary Fig. S4c–e ). The MGAT1 IV A V T−T haplotype also limited CTLA-4 surface levels when expressed with the common CTLA- 4 Thr17 allele (two N -glycans) whereas combining the MGAT1 IV A V T−T haplotype with CTLA-4 Ala17 (one N -glycan) further reduced CTLA-4 surface levels. These phenotypes were rescued by increasing UDP-GlcNAc levels and/or GlcNAc supplementation, confirming that these phenotypes are sensitive to metabolism. GlcNAc also inhibited proliferation of T cells heterozygous for the MGAT1 IV A V T−T haplotype ( Supplementary Fig. S4f ). Soluble receptors associated with the IL2RA *T and IL7RA *C MS risk alleles reduce Mgat1 mRNA and should interact with Mgat1 upregulation by the MGAT1 IV A V T−T haplotype to control branching ( Fig. 4a ). Indeed, addition of exogenous IL-2 or IL-7 enhanced branching in control cells but reduced branching in MGAT1 IV A V T−T heterozygous cells ( Fig. 4e , interaction P =1.7×10 −5 ). These results were predicted by computational modelling, with upregulation of Mgat1 by IL-2 or IL-7 enhancing or reducing branching depending on baseline Mgat1 activity ( Fig. 4a ). Taken together, these data indicate that the MGAT1 IV A V T−T haplotype lowers branching, T cell activation thresholds and CTLA-4 surface retention in a manner that is sensitive to metabolic conditions (that is, UDP-GlcNAc), activity of other Golgi branching enzymes (for example, Mgat5), the number of N -glycans attached to CTLA-4 (that is, CTLA-4 Thr17Ala) and IL-2 and IL-7 signalling. Genetic interactions in MS The biological interactions defined above for IL2RA (rs2104286), IL7RA (rs6897932), MGAT1 IV A V T−T (rs7726005, rs2070924 and rs2070925) and CTLA-4 Thr17Ala (rs231775) are expected to result in genetic interaction in MS. To test this hypothesis, we first examined point association of the four variants in two Caucasian MS case–control cohorts from North America ( n =2,705 and n =9,132, respectively). We replicated association of IL2RA (rs2104286) and IL7RA (rs6897932) as well as the lack of association of CTLA-4 (rs231775) in both cohorts ( Table 1 , Supplementary Table S1 ) [3] , [22] , [23] , [34] . Although the MGAT1 IV A V T−T haplotype is relatively rare (carrier frequency ∼ 7.2%), we observed a novel association for carrier status in both cohorts, with P =1.51×10 −5 and odds ratio (OR)=1.36 in combined data of 3,280 cases and 8,557 controls ( Table 1 , Supplementary Table S1 ). Allelic analysis yielded a trend P value (Cochran–Armitage) of 1.90×10 −5 (1 tail) for combined data. Pearson's correlation ( r ) confirmed that the IV A (rs7726005) and V T−T (rs2070924 and rs2070925) polymorphisms are in strong linkage disequilibrium ( r =0.633695, P <2.2×10 −16 ), as first observed by physical cloning and sequencing of genomic DNA ( Fig. 3a ). Analysis of the IV A and V T–T polymorphisms irrespective of haplotype revealed association of V T–T (rs2070924 and rs2070925; P =1.67×10 −4 , OR=1.29) and marginal association of IV A (rs7726005, P =1.66×10 −2 , OR=1.13 ( Supplementary Table S1 )). Table 1 Genetic interaction in multiple sclerosis. Full size table As gene–gene interaction analysis requires large sample sizes (power calculations in Table 1 ), especially when alleles are rare, we conducted stratified analysis in both Caucasian cohorts and interaction analyses only in combined data. Consistent with opposing effects on Mgat1 that optimize enzyme activity and branching when combined, stratified analysis of the Caucasian data reveals that MGAT1 IV A V T−T significantly increases MS risk when there are less than four copies of the IL2RA *T and IL7RA *C risk alleles ( P =3.60×10 −5 , OR=1.45), whereas no association was observed in the presence of four copies of the IL2RA *T and IL7RA *C ( P =0.195, OR=1.13; Table 1 , Supplementary Table S2 ). The P value for interaction is 6.75×10 −2 . Next, we tested for interaction of MGAT1 IV A V T−T with CTLA-4 Thr17Ala (rs231775). CTLA-4 Thr17 harbours twice as many N -glycans as CTLA-4 Ala17 and therefore should compensate for reduced branching by MGAT1 IV A V T−T to mitigate MS risk. Indeed, MGAT1 IV A V T−T significantly associated with MS in CTLA-4 Ala17 carriers ( P =4.95×10 −6 , OR=1.53), but not CTLA-4 Thr/Thr homozygotes ( P =0.329, OR=1.06) with an interaction P value of 1.20×10 −2 ( Table 1 , Supplementary Table S2 ). Stratifying the data based on six or less than six alleles of CTLA-4 Thr17, IL2RA *T and IL7RA *C strengthened the interaction, with MGAT1 IV A V T−T -promoting MS in the latter ( P =1.62×10 −6 , OR=1.46), whereas appearing to be protective in the former ( P =4.08×10 −2 , OR=0.64), giving an interaction P value of 9.48×10 −4 . Finally, we examined an independent African-American MS cohort (758 cases, 480 controls). On the basis of HapMap data, IL2RA *T and IL7RA *C risk alleles are much more common in Sub-Saharan Africans/African-Americans (risk allele frequencies of ∼ 0.90–0.95 versus ∼ 0.75 in Caucasians). Indeed, analysis of a subset of the African-American MS cases ( n =478) revealed IL2RA *T and IL7RA *C allele frequencies of 0.94 and 0.88, respectively. As these high frequencies limit power, we restricted further analysis of the African-American cohort to MGAT1 IV A V T−T and CTLA-4 Thr17Ala. MGAT1 IV A V T−T did not display association in African-American MS ( P =0.215), with an OR similar to Caucasians with IL2RA *T + IL7RA *C=4 (that is, 1.15 versus 1.13, respectively), a result consistent with the much higher frequencies of IL2RA *T and IL7RA *C in African-Americans ( Table 1 ). However, stratifying the data based on CTLA-4 Thr17Ala replicated the Caucasian MS data, with MGAT1 IV A V T−T -promoting MS in CTLA-4 Ala17 carriers ( P =8.40×10 −3 , OR=1.82), but appearing to be protective in CTLA-4 Thr/Thr homozygotes ( P =4.95×10 −2 , OR=0.64), with an interaction P value of 2.29×10 −3 . The OR in CTLA-4 Thr/Thr homozygotes is similar to that in Caucasians with six alleles of CTLA-4 Thr17, IL2RA *T and IL7RA *C (that is, 0.64 and 0.64, respectively), again consistent with the much higher frequencies of IL2RA *T and IL7RA *C in African-Americans. Combining the African-American and Caucasian P values gives P =7.48×10 −7 for CTLA-4 Ala17 carriers and P =3.16×10 −4 for interaction. Importantly, this interaction is observed despite lack of point association and marginal effects of CTLA-4 Thr17Ala in both the Caucasian and African-American data, indicating an epistatic interaction. Thus, the Caucasian and African-American MS data are concordant and when combined with the demonstrated biological interactions, provide strong evidence that the four variants converge on N -glycosylation to differentially regulate MS risk. Vitamin D 3 enhances Mgat1 to inhibit demyelinating disease Deficiency of vitamin D 3 , which is synthesized from 7-dehydrocholesterol in the skin on ultraviolet sun exposure, strongly associates with MS [2] , [35] , [36] . Vitamin D 3 and/or its active metabolite 1α,25-dihydroxyvitamin D 3 (1,25(OH) 2 D 3 ) inhibit T cell activation [37] , interferon-γ production [38] and T cell-mediated demyelinating disease [38] ; however, molecular mechanisms are unclear. 1,25(OH) 2 D 3 enhanced MGAT1 mRNA levels in human male and female CD4 + CD25 + T cell blasts, a phenotype similar to the MGAT1 IV A V T−T haplotype but opposite of the IL2RA *T+ IL7RA *C risk alleles ( Fig. 5a ). 1,25(OH) 2 D 3 also increased MAN1A1 , but had little effect on other Golgi branching genes. In the presence of the IL2RA* T and IL7RA* C risk alleles, 1,25(OH) 2 D 3 should enhance branching by reversing Mgat1 downregulation resulting from reduced IL-2 and IL-7 signalling. In contrast, upregulation of Mgat1 by 1,25(OH) 2 D 3 in T cell blasts lacking the IL2RA* T and IL7RA* C risk alleles is expected to have little or negative effect. Indeed, although 1,25(OH) 2 D 3 enhanced branching in T cell blasts with two or more copies of the IL2RA* T and IL7RA* C risk alleles ( Fig. 5b ), branching was unchanged or reduced (depending on TCR stimulation strength) in blasting T cells homozygous for both protective alleles ( Fig. 5c and Supplementary Fig. S5 ). Addition of exogenous sIL2RA and sIL7RA to the latter cells, thereby mimicking the IL2RA* T and IL7RA* C risk alleles, restored the ability of 1,25(OH) 2 D 3 to enhance branching ( Fig. 5c ). As a very small minority of Caucasians are homozygous for the IL2RA* C and IL7RA* T protective alleles ( ∼ 0.5%), vitamin D 3 is expected to promote branching in the majority of the population. 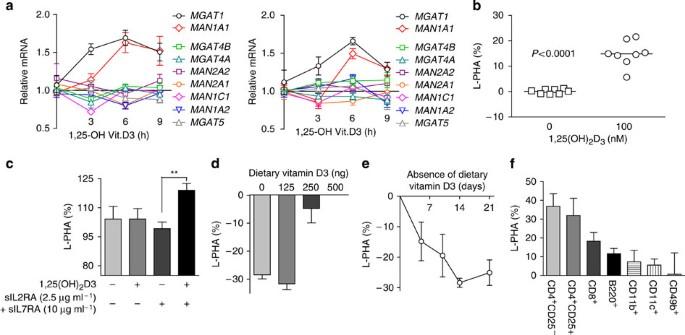Figure 5: Vitamin D3countersIL2RA*T- andIL7RA*C-mediated reduction in Mgat1 to promoteN-glycan branching. (a) Male (right) or female (left) purified human CD4+T cells were pre-stimulated with plate-bound anti-CD3 for 4 days (1 μg ml−1) then treated with 100 nM 1,25(OH)2D3for 3, 6 and 9 h. Blasting CD25+T cells were isolated and collected for mRNA extraction and cDNA synthesis. Relative mRNA levels of indicated genes were performed by quantitative reverse transcription PCR analysis and normalized to actin. (b) Human CD3+T cells harbouring two or moreIL2RA*T+IL7RA*Crisk alleles (that is,IL2RA*T+IL7RA*C≥2) were pre-stimulated with anti-CD3 for 2 days (1 μg ml−1) then treated with 100 nM 1,25(OH)2D3for 3 days before fluorescence-activated cell sorting (FACS) analysis forL-PHA binding in CD4+cells. All donors are negative forMGAT1IVAVT−T. Horizontal bar represents the averageL-PHA MFI of each treatment group. (c) Human CD3+T cells lacking theIL2RA*T andIL7RA*C risk alleles (that is,IL2RA*T+IL7RA*C=0, common haplotype forMGAT1) were pre-stimulated with anti-CD3 (400 ng ml−1) and pre-treated with sIL2RA/sIL7RA for 2 days before addition of 100 nM 1,25(OH)2D3for another 3 days.L-PHA binding was analysed as inb.Pvalue byt-test. **P<0.01. (d) PL/J mice were fed 4 g per day of chow containing varying amounts of vitamin D3for 14 days. Splenocytes were isolated and analysed forL-PHA binding in CD4+T cells as inb. Two mice (n=2) for each group with each mouse stained in triplicate. Error bars represent the range of biological replicates (e) PL/J mice were maintained on either a regular mouse diet obtaining∼500–625 ng vitamin D3per day or on a diet deficient in vitamin D3for the indicated number of days. Splenocytes were collected and analysed as ind.n=6 andn=4 mice per time point for the first and last two times points, respectively, with each mouse stained in triplicate. Error bars represent the range of biological replicates. (f) Mice consuming∼500–625 ng dietary vitamin D3per day were injected with 100 ng 1,25(OH)2D3by intraperitoneal injection every other day for a total of three times. Splenocytes were collected 24 h after the last injection and analysed forL-PHA binding in the indicated cell types by FACS.n=8 mice stained in triplicate with error bars representing standard error of biological replicates. CD11b+, macrophages; CD11c+, dendritic cells; CD49b+, NK cells; Error bars are standard error of triplicate or greater values unless otherwise stated. Figure 5: Vitamin D 3 counters IL2RA *T- and IL7RA *C-mediated reduction in Mgat1 to promote N -glycan branching. ( a ) Male (right) or female (left) purified human CD4 + T cells were pre-stimulated with plate-bound anti-CD3 for 4 days (1 μg ml −1 ) then treated with 100 nM 1,25(OH) 2 D 3 for 3, 6 and 9 h. Blasting CD25 + T cells were isolated and collected for mRNA extraction and cDNA synthesis. Relative mRNA levels of indicated genes were performed by quantitative reverse transcription PCR analysis and normalized to actin. ( b ) Human CD3 + T cells harbouring two or more IL2RA*T + IL7RA*C risk alleles (that is, IL2RA* T+ IL7RA* C≥2) were pre-stimulated with anti-CD3 for 2 days (1 μg ml −1 ) then treated with 100 nM 1,25(OH) 2 D 3 for 3 days before fluorescence-activated cell sorting (FACS) analysis for L -PHA binding in CD4 + cells. All donors are negative for MGAT1 IV A V T−T . Horizontal bar represents the average L -PHA MFI of each treatment group. ( c ) Human CD3 + T cells lacking the IL2RA* T and IL7RA* C risk alleles (that is, IL2RA* T+ IL7RA* C=0, common haplotype for MGAT1 ) were pre-stimulated with anti-CD3 (400 ng ml −1 ) and pre-treated with sIL2RA/sIL7RA for 2 days before addition of 100 nM 1,25(OH) 2 D 3 for another 3 days. L -PHA binding was analysed as in b . P value by t -test. ** P <0.01. ( d ) PL/J mice were fed 4 g per day of chow containing varying amounts of vitamin D 3 for 14 days. Splenocytes were isolated and analysed for L -PHA binding in CD4 + T cells as in b . Two mice ( n =2) for each group with each mouse stained in triplicate. Error bars represent the range of biological replicates ( e ) PL/J mice were maintained on either a regular mouse diet obtaining ∼ 500–625 ng vitamin D 3 per day or on a diet deficient in vitamin D 3 for the indicated number of days. Splenocytes were collected and analysed as in d . n =6 and n =4 mice per time point for the first and last two times points, respectively, with each mouse stained in triplicate. Error bars represent the range of biological replicates. ( f ) Mice consuming ∼ 500–625 ng dietary vitamin D 3 per day were injected with 100 ng 1,25(OH) 2 D 3 by intraperitoneal injection every other day for a total of three times. Splenocytes were collected 24 h after the last injection and analysed for L -PHA binding in the indicated cell types by FACS. n =8 mice stained in triplicate with error bars representing standard error of biological replicates. CD11b+, macrophages; CD11c+, dendritic cells; CD49b+, NK cells; Error bars are standard error of triplicate or greater values unless otherwise stated. Full size image T cells from the PL/J mouse strain are deficient in Mgat1 activity (that is, ∼ 3.3 versus 5.57 nmol mg −1 h −1 in 129/Sv) and branching [20] , providing a model for Mgat1 deficiency similar to the IL2RA *T and IL7RA *C MS risk alleles. The vitamin D 3 receptor is minimally expressed in naive ex vivo T cells and upregulated by TCR or vitamin D 3 signalling [39] . Addition of 1,25(OH) 2 D 3 to resting PL/J mouse or human T cells had little affect on branching ( Supplementary Fig. S6a,b ), whereas addition to TCR-activated female PL/J mouse T cells enhanced branching ( Supplementary Fig. S6c ). Consistent with previous observations that 1,25(OH) 2 D 3 inhibits experimental autoimmune encephalomyelitis (EAE) in C57BL/6 female but not male mice, 1,25(OH) 2 D 3 had minimal effects on branching in male PL/J mouse T cell blasts ( Supplementary Fig. S6d ); however, both male and female human T cell blasts responded similarly with enhanced branching ( Supplementary Fig. S6e,f ). C57BL/6 mice are also deficient in Mgat1 activity, however, branching is reduced to a much smaller degree than PL/J mice [20] . Reducing dietary supply of vitamin D 3 in female PL/J mice decreased branching in CD4 + T cells in vivo in a dose- and time-dependent manner ( Fig. 5d,e ). Intraperitoneal injection of 1,25(OH) 2 D 3 in female PL/J mice enhanced branching in CD4 + T cells > CD8 + T cells > B cells (B220 + ) but had little effect in CD11b + cells (macrophages), CD11c + cells (dendritic cells) or CD49b + cells (NK cells; Fig. 5f ). Blocking branching with SW reversed 1,25(OH) 2 D 3 -induced T cell hypoproliferation in response to TCR stimulation ( Fig. 6a ). 1,25(OH) 2 D 3 enhanced CTLA-4 cell surface expression in PL/J mouse and human T cell blasts ( Fig. 6b and Supplementary Fig. S7a,b ) and markedly reduced CTLA-4 endocytosis rates ( Fig. 6c ). Intraperitoneal injection of 1,25(OH) 2 D 3 inhibited myelin basic protein (MBP)-induced EAE in PL/J female mice in the absence but not presence of SW in the drinking water ( Fig. 6d ), where SW reduced branching in CD4 + T cells ∼ 50% ( Supplementary Fig. S7c ). SW also reversed 1,25(OH) 2 D 3 -induced hypoproliferation in MBP-stimulated T cells isolated from MBP-immunized PL/J mice ( Fig. 6e ). Thus, vitamin D 3 promotes branching and CTLA-4 surface retention to suppress T cell growth and autoimmune demyelinating disease when Mgat1 activity is suppressed, as occurs with the IL2RA* T and IL7RA* C risk alleles and in the C57BL/6 and PL/J mouse strains. 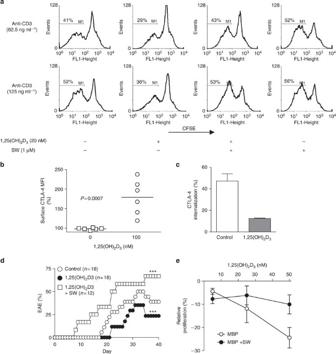Figure 6: Vitamin D3regulates T cell growth and EAE. (a) Purified mouse CD3+T cells were stained with CFSE, stimulated with plate-bound anti-CD3 antibody in the presence or absence of 1,25(OH)2D3(20 nM) for 3 days and analysed by fluorescence-activated cell sorting (FACS) for CFSE dilution/proliferation in CD4+T cells. Horizontal bars mark the population of proliferating cells, with the percentage of proliferating cells noted above. (b) Purified human CD3+T cells (n=8 donors per group) were pre-stimulated with plate-bound anti-CD3 for 2 days (1 μg ml−1) then treated with 100 nM 1,25(OH)2D3for 3 days. CD25+CD4+blasting T cells were analysed for surface CTLA-4 expression by FACS. Horizontal bar represents the averageL-PHA MFI of each treatment group.Pvalue determined byt-test. (c) Purified mouse CD3+T cells were stimulated with plate-bound anti-CD3 (250 ng ml−1) in the presence or absence of 1,25(OH)2D3(150 nM) for 5 days and analysed by FACS for internalization rates of cell surface CTLA-4 in CD4+T cells. (d) PL/J mice treated as indicated were immunized with MBP+CFA and examined daily for clinical EAE. 1,25(OH)2D3of 100 ng was administered by intraperitoneal injection every other day starting at day −3. SW was provided in drinking water and reducedL-PHA staining∼50%.Pvalues by Fisher's exactt-test, ***P<0.0001. (e) Female mice were immunized with 100 μg MBP+CFA by intraperitoneal injection and after 10 days, splenocytes were collected and re-stimulatedin vitrowith MBP in the presence or absence of 1,25(OH)2D3and/or SW as indicated. Proliferation was assessed by CFSE dilution and analysed by FACS. Error bars are standard error of triplicate or greater values in all panels. Figure 6: Vitamin D 3 regulates T cell growth and EAE. ( a ) Purified mouse CD3 + T cells were stained with CFSE, stimulated with plate-bound anti-CD3 antibody in the presence or absence of 1,25(OH) 2 D 3 (20 nM) for 3 days and analysed by fluorescence-activated cell sorting (FACS) for CFSE dilution/proliferation in CD4 + T cells. Horizontal bars mark the population of proliferating cells, with the percentage of proliferating cells noted above. ( b ) Purified human CD3 + T cells ( n =8 donors per group) were pre-stimulated with plate-bound anti-CD3 for 2 days (1 μg ml −1 ) then treated with 100 nM 1,25(OH) 2 D 3 for 3 days. CD25 + CD4 + blasting T cells were analysed for surface CTLA-4 expression by FACS. Horizontal bar represents the average L -PHA MFI of each treatment group. P value determined by t -test. ( c ) Purified mouse CD3 + T cells were stimulated with plate-bound anti-CD3 (250 ng ml −1 ) in the presence or absence of 1,25(OH) 2 D 3 (150 nM) for 5 days and analysed by FACS for internalization rates of cell surface CTLA-4 in CD4 + T cells. ( d ) PL/J mice treated as indicated were immunized with MBP+CFA and examined daily for clinical EAE. 1,25(OH) 2 D 3 of 100 ng was administered by intraperitoneal injection every other day starting at day −3. SW was provided in drinking water and reduced L -PHA staining ∼ 50%. P values by Fisher's exact t -test, *** P <0.0001. ( e ) Female mice were immunized with 100 μg MBP+CFA by intraperitoneal injection and after 10 days, splenocytes were collected and re-stimulated in vitro with MBP in the presence or absence of 1,25(OH) 2 D 3 and/or SW as indicated. Proliferation was assessed by CFSE dilution and analysed by FACS. Error bars are standard error of triplicate or greater values in all panels. Full size image Defining how environmental factors combine with genetic risk at the molecular level to promote complex trait diseases such as MS has remained a great challenge. Here we suggest a unifying molecular mechanism in MS, whereby multiple environmental factors (sunlight/vitamin D 3 and metabolism) converge with multiple genetic variants ( IL-7RA , IL-2RA , MGAT1 and CTLA-4 ) to dysregulate a final common pathway, Golgi N -glycosylation ( Fig. 7 ). A causal role for defective N -glycosylation is supported by the development of spontaneous inflammatory demyelination and neurodegeneration in Mgat1 and/or Mgat5-deficient mice [17] , [20] , as well as the observed biological and genetic interactions that appear to differentially control N -glycosylation and MS risk. The ability of environmental factors such as vitamin D 3 /sunshine and/or metabolism to directly compensate for genetic downregulation of branching is consistent with concordance rates in monozygotic twins of only ∼ 30% and their lack of significant detectable genomic, epigenomic or transcriptome differences [10] , [11] . Therapeutic supplementation to N -glycan biosynthesis may serve as a simple therapy to suppress phenotypic expression of MS risk factors. Indeed, vitamin D 3 (1,25(OH) 2 D 3 ) and GlcNAc are orally active, rescue branching deficiency on mouse T cells in vivo and inhibit EAE and spontaneous autoimmune diabetes in mice [16] , [38] , [40] . In humans, oral GlcNAc improved disease in 8 of 12 children with treatment-resistant inflammatory bowel disease [41] . 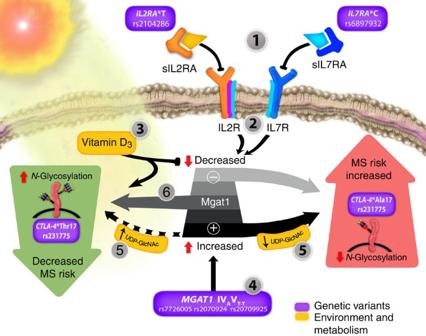Figure 7: A model for environmental and genetic dysregulation ofN-glycosylation in multiple sclerosis. Environmental and genetic interaction converges on the GolgiN-glycan branching enzyme Mgat1 andN-glycosylation of CTLA-4 in T cell blasts. Both down- or upregulation of Mgat1 activity decrease branching by limitingN-glycan or UDP-GlcNAc substrate to downstream enzymes, respectively. (1) Soluble receptors associated with theIL2RA*T (rs2104286) andIL7RA*C (rs6897932) MS risk alleles antagonize IL-2 and IL-7 signalling, leading to (2) downregulation of Mgat1, decreased branching and CTLA-4 surface levels and increased MS risk. (3) Vitamin D3 signalling counteracts this by enhancing Mgat1, leading to increased branching, CTLA-4 surface expression and decreased MS risk. (4) TheMGAT1IVAVT–T haplotype (rs7726005, rs2070924, rs2070925) increases Mgat1, which decreases branching, CTLA-4 surface levels and increases MS risk conditional on (5) metabolic production of UDP-GlcNAc. (6) Combining genetic upregulation of Mgat1 by theMGAT1IVAVT–T haplotype with genetic downregulation of Mgat1 by theIL2RA*T andIL7RA*C MS risk alleles optimizes Mgat1 activity, thereby enhancing branching, CTLA-4 surface expression and mitigating MS risk. TheCTLA-4Thr17Ala (rs231775) variant modifies these interactions by controlling the number ofN-glycans attached to CTLA-4, with the Thr17 allele doublingN-glycan number to promote CTLA-4 surface retention and reduce MS risk when combined withMGAT1IVAVT–T,IL2RA*TT andIL7RA*CC. Figure 7: A model for environmental and genetic dysregulation of N -glycosylation in multiple sclerosis. Environmental and genetic interaction converges on the Golgi N -glycan branching enzyme Mgat1 and N -glycosylation of CTLA-4 in T cell blasts. Both down- or upregulation of Mgat1 activity decrease branching by limiting N -glycan or UDP-GlcNAc substrate to downstream enzymes, respectively. (1) Soluble receptors associated with the IL2RA *T (rs2104286) and IL7RA *C (rs6897932) MS risk alleles antagonize IL-2 and IL-7 signalling, leading to (2) downregulation of Mgat1, decreased branching and CTLA-4 surface levels and increased MS risk. (3) Vitamin D3 signalling counteracts this by enhancing Mgat1, leading to increased branching, CTLA-4 surface expression and decreased MS risk. (4) The MGAT1 IVAVT–T haplotype (rs7726005, rs2070924, rs2070925) increases Mgat1, which decreases branching, CTLA-4 surface levels and increases MS risk conditional on (5) metabolic production of UDP-GlcNAc. (6) Combining genetic upregulation of Mgat1 by the MGAT1 IVAVT–T haplotype with genetic downregulation of Mgat1 by the IL2RA *T and IL7RA *C MS risk alleles optimizes Mgat1 activity, thereby enhancing branching, CTLA-4 surface expression and mitigating MS risk. The CTLA-4 Thr17Ala (rs231775) variant modifies these interactions by controlling the number of N -glycans attached to CTLA-4, with the Thr17 allele doubling N -glycan number to promote CTLA-4 surface retention and reduce MS risk when combined with MGAT1 IVAVT–T, IL2RA *TT and IL7RA *CC. Full size image Defective N -glycosylation likely promotes MS by multiple mechanisms. Reduced N -glycosylation lowers T cell activation thresholds and surface expression of the autoimmune inhibitor CTLA-4, promoting loss of self-tolerance. Mgat1 dysfunction may expose cryptic mannose linkages on the cell surface of oligodendrocytes that mimic microbial and pathogen glycans, chronically activating innate immune responses [42] , [43] . Neurodegeneration in MS may arise from increased sensitivity to apoptotic stimuli. Indeed, targeted deficiency of Mgat1 in neurons induces their apoptosis in vivo , whereas Mgat5 deficiency enhances spontaneous neurodegeneration along with inflammatory demyelination [17] , [20] . Thus, genetic and environmental alterations in the N -glycosylation pathway likely synergize to promote MS through dysfunction of both immune (T cells, antigen presenting cells) and target cells (oligodendrocytes, neurons). IL2RA* T (rs2104286), IL7RA* C (rs6897932) and vitamin D 3 deficiency also associate with type 1 diabetes (T1D) [28] , [44] , [45] , [46] , whereas non-obese diabetic mice are deficient for branching in T cells but not B cells [20] . A second independent variant of IL2RA (rs11594656) also alters sIL2RA levels and associates with both MS and T1D [28] , but paradoxically in opposite directions. CTLA-4 Ala17 (rs231775) displays point association with T1D but not MS [34] , [47] . These considerations imply that defective N -glycosylation likely also contributes to T1D risk; however, interactions between these variants and MGAT1 IV A V T−T may differ because of disparity in CTLA-4 Ala17 (rs231775) frequencies between T1D and MS. Direct affects of branching deficiency on neuronal survival would also be expected to result in distinctive interactions in MS compared with T1D and other autoimmune diseases. IL-7 and IL-2 both promote T cell growth, yet targeted deficiencies of these pathways in mice induce immunodeficiency and spontaneous autoimmunity, respectively [48] , [49] . Our data suggest that by having opposing effects on branching in resting and activated T cells, IL-2 and IL-7 enhance T cell growth early by lowering branching and TCR activation thresholds but promote self-tolerance later by enhancing branching and CTLA-4 surface retention. Before GWAS, many candidate gene studies proved unreliable. This failure likely arose from multiple issues such as very small sample size, lack of replication cohorts, poor selection of candidate genes (that is, no evidence for regulating spontaneous disease in animals) and association testing in the absence of detailed functional characterization. We avoided these issues by initially ignoring association testing and performing a detailed biological screen for functional variants that induce phenotypes causal of disease in mice. Critically, only the single variant with the greatest biological effect is selected for subsequent association testing in large cohorts. This reverse approach also avoids the problem of multiple hypothesis testing inherent to GWAS. Indeed, the P values we report ( ∼ 10 −5 to 10 −7 ) are orders of magnitude better than the genome-wide significance level of ∼ 5×10 −8 that corrects to ∼ 0.02 after adjusting for multiple hypothesis testing in a typical GWAS with ∼ 550,000 SNPs [50] . As the N -glycan branching pathway includes at least ∼ 30 genes likely to also harbour variants that alter branching, the additive risk reported here probably underestimates the true magnitude of genetic dysregulation of N -glycosylation in MS. Indeed, the top hit in a recent GWAS for variants regulating disease severity in MS was MGAT5 (ref. 51 ). More broadly, our data suggest an alternative to the rare allele—common disease hypothesis by implicating genetic and environmental interaction of common factors that additively converge to disrupt a critical biochemical pathway regulating disease. Reagents and flow cytometry Isolated PBMCs (Histopaque-1077; Sigma) were stimulated with soluble anti-CD3 (Biomeda). CD3 + T cells purified by negative selection (RosetteSep, StemCell Technologies) were stimulated with plate-bound anti-CD3 (OKT3, eBioscience). CD25 + cells were positively selected by EasySep (StemCell Technologies). Procedures with human subjects were approved by the Institutional Review Board of the University of California, Irvine. IL-2 (stock#002252) and IL7RA (stock#002295) deficient mice (Jackson Laboratories) were used between 4 and 8 weeks of age. IL7R −/− Mgat5 −/− mice were obtained by crossing IL7RA-deficient mice with C57BL/6 Mgat5 −/− mice. All mice were selected randomly for experiments and approved by the Institutional Animal Care and Use Committee of the University of California, Irvine. IL2RA antagonist Ro26-4550 (Calbiochem), anti-IL-2 (clone#5334), anti-IL-7 (clone#7417), rhIL2, rhIL7, sIL2RA, sIL7RA/Fc (R&D systems) and rmIL-2 (eBioscience) were used. Human cells were stained with anti-CD4, anti-CTLA-4, anti-CD69 (eBioscience) and/or L -PHA-FITC ( Phaseolus Vulgaris Leukoagglutinin, Vector Labs) as previously described [15] , [16] , [20] . Intracellular pStat5 staining used anti-Stat5pY694 (BDPharmingen, clone#47). Mouse cells were stained with anti-CD4 (RM 4-5), anti-CD8 (53-6.7), anti-CTLA-4 (UC10-4B9), anti-CD69 (H1.2F3), anti-B220 (RA3-6B2), anti-CD11b (M1/70), anti-CD11c (N418) and anti-CD49b (DX5) (eBioscience). Proliferation was assessed by 3H-thymidine incorporation or 5,6-carboxyfluorescein diacetate succinimidyl ester (CFSE; Molecular Probes) at 1 μM in PBS (20 min, 4 °C) and stimulated with plate-bound anti-CD3e (2C11, eBioscience). Cells were cultured in RPMI-1640 media supplemented with 10% fetal bovine serum, 2 μM L -glutamine, 100 U ml −1 penicillin/streptomycin and 2 μM 2-mercaptoethanol. For CTLA-4 internalization, cells were stained for surface CTLA-4 (30 min, 4 °C), washed, incubated at 37 °C at indicated times, washed in cold fluorescence-activated cell sorting buffer or acid for 4 min (0.133 M citric acid, 0.0666 M sodium carbonate, pH3.3). % internalization=100×(mean fluorescence intensity (MFI) acid wash/MFI PBS wash). Quantitative real-time PCR and differential allelic expression RNA from transfected Lec1 cells and human PBMCs/T cells isolated by RNeasy kit (Qiagen) were reverse-transcribed by M-MLV Reverse Transcriptase (Ambion) and analysed by real-time PCR using TaqMan Gene Expression Assays with MGAT1 (Hs00159121_m1), MGAT4a (Hs00923412_m1), MGAT4b (Hs00365001_m1), MGAT5 (Hs00159136_m1), MAN1A1 (Hs00195458_m1), MAN1A2 (Hs00198611_m1), MAN1C1 (Hs00220595_m1), MAN2A1 (Hs00159007_m1), MAN2A2 (Hs00196172_m1), GAPDH (Hs9999905_m1), and ACTIN (Hs99999903_m1) primers (Applied Biosystems). Relative mRNA expression was determined by ΔΔ C t method and normalized for GAPDH or ACTIN expression. Differential allelic expression was performed using two competing TaqMan probes targeting the common and V T–T polymorphisms of MGAT1 in cDNA and genomic DNA isolated from two individuals heterozygous for MGAT1 IV A V T–T haplotype. Reference curves for analysing allelic ratios were generated using plasmid containing either common or V T–T haplotype. DNA sequencing and SNP analysis Exon2 of MGAT , including ∼ 20–100 nucleotides (nt) of intronic sequence at 5′ and 3′ ends, was PCR-amplified from genomic DNA isolated from PBMCs and sequenced by Seqwright. SNPs were identified from chromatograms and derived sequences. All previously unknown SNPs were sequenced in both directions at least once, and confirmed with TaqMan allelic discrimination assay (Applied Biosystems). SNP genotyping was performed using TaqMan Genotyping Assays (Applied Biosystems), except for the controls from the greater Toronto area, which used the Sequenom Mass Array platform for genotyping the two SNPs in MGAT1 V T−T (rs2070924 and rs2070925). These two MGAT1 V T−T SNPs are 10nt apart and were genotyped in all other cohorts using a custom TaqMan probe designed to detect both (sequence submitted to Applied Biosystems was 5′-CCTCGCCCGCGTCTACGGTGCTCCCCAGCTGCAGGTGGAGAAAGTGAGGACCAATGACCGGAAGGAG[C/T]TGGGGGAGGT[G/T]CGGGTGCAGTATACGGGCAGGGACAGCTTCAAGGCTTTCGCCAAGGCTCTGGGTGTCATGGATGACCTTAAGTCGGGGGTTCCGAGAG-3′). MGAT1 IV A (rs7726005) was also genotyped using a custom TaqMan probe (sequence: 5′-CACTACCGCTGGGCGCTGGGCCAGGTCTTCCGGCAGTTTCGCTTCCCCGCGGCCGTGGTGGTGGAGGATGACCTGGAGGTGGCCCCGGACTTCTTCGAGTACTTTC[G/A]GGCCACCTATCCGCTGCTGAAGGCCGACCCCTCCCTGTGGTGCGTCTCGGCCTGGAATGACAACGGCAAGGAGCAGATGGTGGACGCCAGCAGGCCTGAGCTGCTCTA-3′). Accuracy of the custom TaqMan assays was confirmed by sequencing genomic DNA from seven subjects genotyped as heterozygous for both IV A and V T−T and sequencing cloned genomic DNA. Moreover, sequenom genotyping of 1,387 subjects for the two separate SNPs in V T−T revealed 100% concordance. Human subjects are defined as positive or negative for MGAT1 IV A V T−T by genotyping IV A and V T−T polymorphisms. TaqMan Genotpying Assay primers for CTLA-4 (rs231775), IL-2RA (rs2104286) and IL-7R (rs6897932) are C___2415786_20, C__16095542_10 and C___2025977_10, respectively. The genotyping success rate for all five SNPs examined was >99% in all cohorts except for IL2RA in control cohort 2 (98.8%). Concordance for duplicate genotyping was determined by re-genotyping all five SNPs in 735 samples and revealed 100% concordance for all SNPs except CTLA-4 (99.46%). Cloning of human MGAT1 and CTLA-4 variants MGAT1 and CTLA-4 variants were cloned into pCMV-Script (Stratagene), which uses human cytomegalovirus immediate early promoter to drive expression in mammalian systems. For MGAT1 , primers 5′-CCCCCATTTCCTCTACCTGT-3′ and 5′-CCCTCCCACTCATCTGCTTTC-3′ were used to PCR-amplify exon2 from genomic DNA of subjects with or without IV A and V T−T polymorphisms followed by sequencing of PCR products. Full-length cDNA clones for CTLA-4 Thr17 and Ala17 from Mammalian Gene Collection ( http://mgc.nci.nih.gov/ ) were subcloned into pCMV vector following PCR amplification with primers 5′-TGAACACCGCTCCCATAAAG-3′ and 5′-CCTCAGCTCTTGGAAATTGAA-3′. Genotypes were confirmed by allelic discrimination assay. Transient transfections Mgat1-defective Lec1 cells (1×10 5 ) seeded 24 h earlier were incubated (5 h, 37 °C) with 3 μg plasmid DNA and 15 μl LIPOFECTAMINE (Invitrogen) serum-free DMEM and cultured for 72 h. Cells were stained with L -PHA-FITC (4 μg ml −1 )±anti-human CTLA-4-PE (eBioscience; 30 min, 4 °C); MFIs determined on L -PHA + population. Enzymatic assays Mgat1 enzyme activity was measured using the synthetic, specific acceptor αMan(1,3)βMan-O(CH2)7CH3 (Toronto Research Chemicals). Avolume of 10 μl cell lysate (0.9% NaCl, 1% Triton X-100, centrifuged 5,000 g , 15 min, 4 °C) was added to 1 mM acceptor, 1 mM [63H]-UDP-GlcNAc (Amersham) in 50 mM MES pH6.5, 0.1 mM GlcNAc and 25 mM AMP in total of 20 μl. Mgat1 reactions containing 5 mM MnCl 2 , were incubated for 1 h and stopped with ice-cold water. Enzyme products were separated from radioactive substrates by binding to 50 mg C18 cartridges (Alltech) preconditioned with methanol rinsing/water washing. Radiolabelled products were eluted directly into scintillation vials with two 0.5 ml aliquots of methanol; radioactivity was determined by liquid scintillation counting. Matrix-assisted laser desorption/ionization–time of flight mass spectroscopy This was done as a service by Glycotechnology Core Facility at University of California, San Diego. PBMCs were lysed with 1% SDS in 100 mM Tris, pH7.4, dialysed to remove SDS, digested with trypsin to generate glycopeptides and treated with PNGaseF to release N -glycans. N -glycans were desialylated by mild acid digestion before permethylation and mass spectroscopy. Monoisotopic peaks were identified using GlycanMass/GlycoMod software. Computational model Computational modelling of Golgi N -glycan processing and lattice-mediated glycoprotein surface retention was previously described [15] . Briefly, biochemical reaction network for N -glycan processing was represented by a series of ordinary differential equations constructed using generalized mass action formulation and generated structures up to a maximum size of tetra-antennary with N -acetyllactosamine and (Galβ1-4GlcNAcβ1-3) 2 extensions. The fraction of each N -glycan type was used to calculate the glycoform fractions of CTLA-4 in a combinatorial manner dependent on number of N -glycosylation sites. Glycoform avidity for galectin lattice is represented as a linear summation of the affinity of each N -glycan, with avidity enhancements as described previously. Vitamin D3 and experimental autoimmune encephalomyelitis To induce in vivo deficiency of vitamin D3, age-matched littermate female PL/J mice were randomly selected and fed 4 g per day of chow containing varying amounts of vitamin D3 (500–625 ng, 250 ng, 125 ng; Prolab RMH 2,500, LabDiet) or a diet deficient in vitamin D3 (0 ng; specially formulated for our laboratory) for 5–21 days. 1,25(OH)2D3 (100 ng) was administered in vivo to age-matched littermate female PL/J mice (fed diet containing 500–625 ng vitamin D3) by intraperitoneal injection every other day for the duration of the study. EAE was induced by subcutaneous immunization of randomly selected female PL/J mice at days 0 and 15 with 100 μg of bovine MBP (Sigma) emulsified in Complete Freund's Adjuvant containing 4 mg ml −1 heat-inactivated Mycobacterium tuberculosis (H37RA;Difco). Mice were examined daily for clinical signs of EAE over the next 40 days with observer blinded to treatment conditions. Mice were scored daily as follows: 0, no disease; 1, loss of tail tone; 2, hindlimb weakness; 3, hindlimb paralysis; 4, forelimb weakness or paralysis and hindlimb paralysis; 5, moribund or dead. All EAE mice were maintained on a diet low in calcium and vitamin D3 (Certified Rodent Diet 5002*, LabDiet). 1,25(OH)2D3 of 100 ng was administered by intraperitoneal injection every other day and SW was given orally via the drinking water starting 3 days before immunization. All mice were housed with 12-h light/dark cycles. DNA datasets We analysed two independent randomly selected non-Hispanic Caucasian MS case–control cohorts and an African-American MS cohort from North America. Cohort 1 cases consisted of unrelated, non-Hispanic Caucasians with clinically definite MS [52] obtained at University of California, Irvine ( n =82) or from across the United States by Multiple Autoimmune Disease Genetics Consortium ( n =176, http://www.madgc.org ) and Accelerated Cure Project for Multiple Sclerosis ( n =943, http://www.acceleratedcure.org ). Controls were unrelated, non-diabetic, non-Hispanic, Caucasians obtained at University of California, Irvine ( n =102) and from across North America by North American Rheumatoid Arthritis Consortium ( n =192, NARAC, http://www.naracdata.org ) and Type1 Diabetes Genetics Consortium ( n =1,199, http://www.t1dgc.org ). Cohort 2 cases were unrelated, non-Hispanic Caucasians with clinically definite MS obtained from across United States by BioServe ( n =1,030, http://www.bioserve.com ) and University of California, San Francisco ( n =1,050). Cohort 2 controls were non-diabetic, non-Hispanic and unrelated Caucasians obtained from across North America (BioServe ( n =2,972), Genetics of Kidneys in Diabetes (GoKinD; n =746, http://www.niddkrepository.org ), NARAC ( n =1,159), UCSF ( n =796) and greater Toronto area ( n =1,387). GoKinD DNA samples were obtained from National Institute of Diabetes and Digestive and Kidney Diseases. The African-American MS cohort has previously been described [53] and comprises 758 unrelated MS patients and 480 unrelated controls. All study participants are self-reported African-Americans, but European ancestry was documented in the majority of individuals based on genotyping of 186 SNPs highly informative for African versus European ancestry. Global estimation of European ancestry using these markers indicated similar mean admixture proportions in cases and controls (21%). Individual and combined control cohorts were in Hardy Weinberg Equilibrium. How to cite this article: Mkhikian, H. et al . Genetics and the environment converge to dysregulate N -glycosylation in multiple sclerosis. Nat. Commun. 2:334 doi: 10.1038/ncomms1333 (2011).